Third-party social evaluation of humans by monkeys Humans routinely socially evaluate others not only following direct interactions with them but also based on others’ interactions with third parties. In other species, ‘eavesdropping’ on third-party interactions is often used to gain information about foraging or mating opportunities, or others individuals’ aggressiveness or fighting ability. However, image scoring for potential cooperativeness is less well studied. Here we ask whether a non-human primate species, tufted capuchin monkeys ( Cebus apella ), socially evaluates humans after witnessing third-party interactions involving a helpful intervention or failure to help. We find that the monkeys accept food less frequently from those who persistently reject another’s requests for help. This negative social evaluation effect is robust across conditions, and tightly linked to explicit refusal to help. Evaluation of potential helpfulness based on third-party interactions may thus not be unique to humans. It is advantageous to be able to make judgements about other individuals’ dispositional traits based on their interactions with third parties. In humans, acting upon information gained through ‘eavesdropping’, ‘image scoring’ or ‘reputation’ [1] starts at an early age. For example, after witnessing an adult either helping or ‘harming’ another adult, 3-year-old children were subsequently more likely to help a third (neutral) adult more that the harmful adult [2] . Indeed, third-party social evaluation may emerge even earlier, as suggested by preferences of young infants for helpful versus hindering non-human agents [3] . The term ‘indirect reciprocity’ has been used by evolutionary biologists to describe how individuals acquire and use information about others’ beneficial acts towards, or exploitation of, third parties when deciding how to subsequently interact with those parties [4] . Assessment of conspecifics’ third-party social bonds and competitive abilities through observation has been described in a wide range of species including primates [5] . Eavesdropping on another species’ behaviour may also confer advantages; examples include responding to another species’ alarm calls or food-related calls [6] , [7] , and assessing the degree of ‘cooperativeness’ of potential cleaning mutualism partners [8] . However, the evaluation of social traits, rather than foraging opportunities, based on other species’ third-party social interactions has received little experimental analysis. Here we show that capuchin monkeys discriminate between humans who behave helpfully towards others and those who do not. Capuchins are noted among primates for their high degree of social tolerance and prosociality, including cooperating on a range of tasks [9] , [10] , [11] , [12] , [13] , [14] . Specifically, monkeys were less likely to accept food from someone who previously refused a request for help from another person. Thus, at least one species of non-human primate is capable of cross-species indirect reciprocity based on interactions that are of no direct relevance to the observer. Helpful versus non-helpful persons For Experiment 1, we tested seven capuchin monkeys. In front of each monkey, two actors performed in ways that portrayed a helpful or a non-helpful disposition. In six ‘helper’ sessions, actor A tried to get a toy out of a container, requested help from actor B, and the latter helped. In six ‘non-helper’ sessions B refused to help ( Fig. 1a ), leaving A to continue in vain. Both actors then offered a piece of food to the monkey, who accepted one offer. 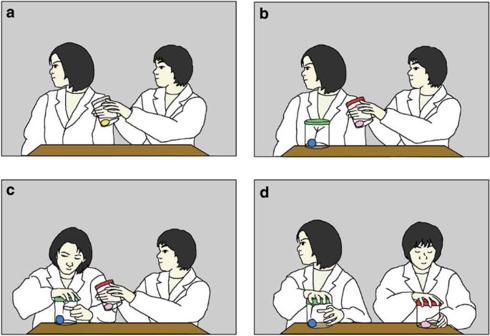Figure 1: Human interactions observed by monkeys. (a) A requests help; B refuses by turning away (Experiment 1). (b) A requests help; B refuses by turning away (Experiment 2); she goes on to manipulate the container in front of her (as inc). (c) A requests help; B does not acknowledge the request but continues to manipulate her container (Experiment 3). (d) Both actors briefly stop manipulating their containers, while B turns away from A; this is not a refusal to help (Experiment 4). In helper sessions, monkeys readily accepted food from both actors, showing no significant bias ( Table 1 ). In contrast, in non-helper sessions they accepted food more frequently from A (attempter) than B (non-helper) (Student’s t -test, t =2.71, df=6, P =0.035). There was no significant correlation between session number and frequency of selecting either actor (Spearman’s rho=0.09, P =0.841), ruling out learning across sessions. Comparing frequency of selecting B in the two types of session confirmed the bias against the non-helper (Student’s t -test, t =−2.51, P =0.046) ( Fig. 2 ). In non-helper sessions, A and B were chosen significantly more than and less than expected by chance, respectively (one-sample t -test, t =2.71, df=6, P =0.035). Figure 1: Human interactions observed by monkeys. ( a ) A requests help; B refuses by turning away (Experiment 1). ( b ) A requests help; B refuses by turning away (Experiment 2); she goes on to manipulate the container in front of her (as in c ). ( c ) A requests help; B does not acknowledge the request but continues to manipulate her container (Experiment 3). ( d ) Both actors briefly stop manipulating their containers, while B turns away from A; this is not a refusal to help (Experiment 4). Full size image Table 1 Individual monkeys’ food acceptance results with the actors playing different roles. 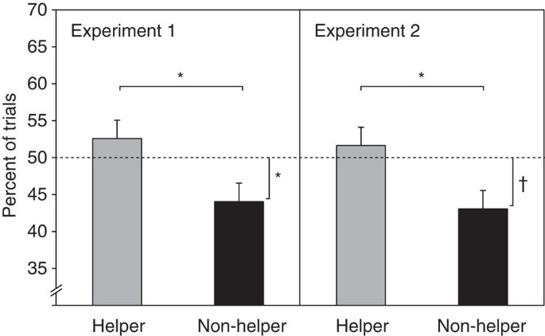Figure 2: Mean frequency of accepting food offered by the helper and the non-helper. Both Experiments 1 and 2 involved the monkeys accepting food from helpers and non-helpers. In Experiment 1,N=7; in Experiment 2,N=6 (see Results). *P<0.05; †P>0.05<0.10. Error bars represent mean±s.e.m. Full size table Figure 2: Mean frequency of accepting food offered by the helper and the non-helper. Both Experiments 1 and 2 involved the monkeys accepting food from helpers and non-helpers. In Experiment 1, N =7; in Experiment 2, N =6 (see Results). * P <0.05; † P >0.05<0.10. Error bars represent mean±s.e.m. Full size image Equalized competence and activity Experiment 2 followed the same general procedure as previously, but now each actor had a container with a small toy inside. At the start of and half-way through each session, we presented ‘success demonstrations’ to show that both actors could open the containers: each actor manipulated a container for 5 s, opened it and emptied the contents into one hand. In helper sessions, B again responded positively to A’s request for help, but their joint manipulation of the container did not result in success. In non-helper sessions, not only did B again refuse to help ( Fig. 1b ), she also began to manipulate her own container, thus equalizing post-request manipulatory activity. In helper sessions, the monkeys again expressed no overall bias towards either actor. In non-helper sessions, the tendency to accept food more often from the attempter than the non-helper was marginally significant (Student’s t -test, t =1.48, df=6, P =0.095); there was again no significant correlation between this measure and session number (Spearman’s rho=0.37, P =0.40). Because one monkey accepted more food from the non-helper in these sessions (Binomial test, P <0.05), we re-ran the analysis excluding this individual; this revealed a significant bias for accepting food from the attempter compared with the non-helper (Student’s t -test, t =2.18, df=5, P =0.046). Direct comparison of frequency of accepting food from B in both conditions confirmed a significant bias against the non-helper (Student’s t -test, t =−2.83, df=5, P =0.019) ( Fig. 2 ). In non-helper sessions, choices of A and B were marginally significantly above and below chance, respectively (one-sample t -test, t =2.14, df=5, P =0.09). Thus, the same tendency to accept food less frequently from the non-helper was observed, albeit less strongly than in Experiment 1. Explicit non-helper versus occupied non-helper In Experiment 3, B did not explicitly refuse to help A, but simply failed to acknowledge A’s request. In these sessions, each actor manipulated a container from the start of the trial. Otherwise, in non-helper sessions B behaved as in Experiment 2 (now called ‘explicit non-helper’ sessions). Helper sessions were replaced by ‘occupied non-helper’ sessions, in which B failed to acknowledge A’s request due to focussing on trying to open her container ( Fig. 1c ). In occupied non-helper sessions, monkeys accepted food non-differentially from the two actors (Student’s t -test, t =−1.64, df=6, P =0.151). In explicit non-helper sessions, there was again a strong bias against the non-helper (Student’s t -test, t =4.60, df=6, P =0.002); the correlation with session number was not significant (Spearman’s rho=0.49, P =0.263). Direct comparison showed that the explicit non-helper was chosen significantly less often than the occupied non-helper (Student’s t -test, t =3.14, df=6, P =0.011) ( Fig. 3 ). In explicit non-helper sessions, A and B were selected more than and less than chance, respectively (one-sample t -test, t =3.14, df=6, P =0.020). 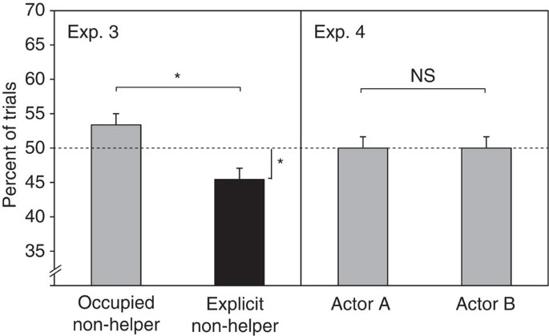Figure 3: Mean frequency of accepting food by different types of non-helpers and non role-playing actors. Experiment 3 involved the monkeys accepting food from an explicit non-helper and an occupied non-helper. Experiment 4 involved accepting food from the actors not playing roles. In both experiments,N=7. *P<0.05. NS, not significant. Error bars represent mean±s.e.m. Figure 3: Mean frequency of accepting food by different types of non-helpers and non role-playing actors. Experiment 3 involved the monkeys accepting food from an explicit non-helper and an occupied non-helper. Experiment 4 involved accepting food from the actors not playing roles. In both experiments, N =7. * P <0.05. NS, not significant. Error bars represent mean±s.e.m. Full size image Controlling for head-turn In a fourth experiment, we examined whether the rejecting non-helper’s gesture of turning away, rather than refusal to help per se , might have led to the expressed discrimination. The materials were as in Experiments 2 and 3. Six sessions were run, each consisting of 2 pairs of success demonstrations and 12 experimental trials as follows: after 5 s of manipulation, A stopped manipulating. While discreetly monitoring A’s activity, B also stopped manipulating and turned away from A for 1–2 s. This movement replicated that shown by B in previous experiments, but now it was not a refusal to help ( Fig. 1d ). As soon as B turned to face forward again, both actors resumed manipulating their containers for 5 s. In these sessions, the mean frequency of accepting offers from A and B was exactly 36 in each case (A range: 33–40) (B range: 32–39), respectively (Student’s t -test, t =0.00, P =1.00 ( Fig. 3 ); indeed, no individual monkey showed a significant bias for either actor. This result rules out any general learning effect across experiments, and the possibility that the simple act of turning away induced a bias in earlier experiments. We conclude that the monkeys’ discriminatory responses required an explicit refusal to help by the non-helper. Overall, capuchins were consistently less willing to accept food from a person of an unhelpful disposition than from a helpful person. The bias against a non-helper persisted across manipulations designed to equate the actors’ activity and competence on the task. In contrast, there was no bias when failure to help was due to the potential helper being occupied with another task, or when there was no request for help. Unlike previous studies in non-humans, the present experimental demonstration of indirect reciprocity in a non-human primate species featured neither food nor dominance-related information in the witnessed social interactions. In an earlier study, chimpanzees spent more time near a human who shared food with another human than one who did not [15] ; this clearly suggests evaluation of a foraging opportunity. Another study reported that chimpanzees begged more from a generous person (who gave another food) than one who withheld food, but only after training [16] ; again this suggests that the apes were interested in getting more food. In the present study, both actors offered identical food to the monkeys; no foraging advantage followed from preferentially accepting food from either actor. In humans, rejecting a gift may signify rejection of the interaction or relationship [17] , [18] ; our data raise the possibility that a similar effect may be seen in other species. It might be asked whether the observed reduced likelihood of accepting food from the non-helper could result from differential attention to the two actors during the demonstration. This seems unlikely for several reasons. First, in the helper condition in Experiment 1 the final action performed by the attempter, namely removing the toy from the container, would have been a recent and salient attention-capturing event, yet it did not influence the monkeys’ selection in the choice phase. Similarly, in Experiments 2–4, container manipulation before the choice phase was comparable between the two actors, but in each case the only factor leading to discrimination by monkeys was the explicit refusal to help by the non-helper. Future studies could incorporate measures of looking behaviour to determine whether visual attention correlates with expressed choice during social evaluation of third-party interactions. Other studies have clearly shown that capuchin monkeys use information gained from watching how humans behave. For example, capuchin monkeys exchanged tokens preferentially with a human who imitated some of their actions, compared with a non-imitator [19] ; in that study, however, no third-party interactions were involved. In another study, capuchins saw a human who previously offered them highly prized food give the same food to a conspecific and then offer them a low-preference alternative [20] . The monkeys often rejected the lower-quality offer. In that example, evaluation was of the rewards, not the human. Here, by contrast, the two actors simultaneously offered food of equal value; the decision which to accept was influenced by the nature of the actors’ behaviour towards each other, not the monkey, and no food was involved in the actors’ interaction with each other. The monkeys consistently showed relative avoidance of explicitly non-helpful individuals, rather than a preference for helpful ones. A negativity bias, reflecting greater saliency of negative as opposed to positive information, is well documented in humans [2] , [21] , including infants as young as 3 months [22] . The present results suggest that a negativity bias exists in other species. Along with work on human infants, they also suggest that such a bias is not a result of teaching. Furthermore, as with human infants [3] , the monkeys’ behaviour was influenced by the intentionality of the refusal to help. When the non-helper’s refusal to help was explicit (Experiments 1 and 2), selective avoidance was evident, but when there was no clear intention to withhold help (Experiments 3 and 4), no discrimination occurred. If capuchins engage in image scoring of humans, as shown here, it seems likely that they also do so in the context of their normal group life with conspecifics. This further suggests that the primate capacity for social evaluation based on third-party interactions might predate the divergence of New World and Old World primates. Alternatively, we might be faced with a case of convergent evolution, with the capacity emerging from the hominoid-like suite of neuroanatomical and psychological traits that characterize capuchin monkeys [9] . Furthermore, the present data raise the possibility that non-human primates may interact with others specifically so as to boost their reputation in the eyes of image scoring third parties [23] . Understanding the evolution of social evaluation processes and their cognitive underpinnings requires more comparative studies; the general approach used here could have a valuable role in such work. Animals The monkeys ( Cebus apella , three males and four females) ranged in age from 6 to 16 years; all were captive-born and group-reared. They were group-housed in a multi-cage complex of over 3 m 2 . They were never food deprived, but earned a portion of their daily intake in a variety of cognitive and social tasks, then received the remainder (commercial primate pellets, fruits, egg, vegetables) every afternoon. They were trained to enter a transport box, and were highly familiar with the test environment and the actors. The were all highly experienced at opening containers to remove contents and had seen humans opening various containers on many occasions. Housing and care of the monkeys adhered to Kyoto University Primate Research Institute’s Guide for the Care and Use of Laboratory Primates (2nd edn). [24] The procedures were approved by the Animal Experiment Committee of the Graduate School of Letters, Kyoto University. Procedure On each trial, an opaque screen was removed to reveal the following scene to monkey: two actors (A and B) sat about 50 cm from the monkey and 25 cm apart. On a table between the actors and monkey was a transparent plastic container (two containers in Experiments 2–4) with a soft toy inside. In Experiment 1, the container was a cuboid, measuring 9 × 9 × 14 cm. In Experiments 2–4, the containers were cylindrical, 10 cm in diameter and 13 cm high; one had a red lid, the other a green lid. In Experiment 1, while B watched, A (the ‘attempter’) manipulated the container, ostensibly trying to open the lid to get the toy. After 5 s of trying, A looked at B and requested help by holding the container towards B. In ‘helper’ sessions, B co-manipulated the container with A for 5 s, reorienting it and thus enabling the latter to remove the lid and get the toy. It was assumed that repeatedly witnessing the request followed by successful co-action would lead to the request–help association being recognized by the monkeys. In ‘non-helper’ sessions when A requested help, B refused to help by turning away for ∼ 2 s, leaving A to continue unsuccessfully for another 5 s. The opaque screen was again interposed between monkey and actors, and the container and toy were placed out of sight below the table. After 5 s, the screen was removed to reveal both actors offering the monkey an identical piece of food, namely a small primate pellet resting between the third and fourth fingers of the hand nearest the midline of the table, palm up. A line across the table served as a marker to ensure that the actors’ hands were the same distance from the screen ( ∼ 10 cm), their hands 5–7 cm apart. The actors maintained a neutral expression and fixated a spot on the table just beyond their fingertips. The monkey extended an arm through a 3-cm gap at the front of the test box to indicate which offer was accepted. The chosen actor then extended the hand and allowed the monkey to take the food while the other actor’s hand withdrew. After the monkey took the food, the screen was again placed in front of the box and the inter-trial interval (ITI) began. ITIs lasted 10–15 s, during which the next trial was prepared. The positions (left or right) of A and B varied pseudo-randomly across trials, so they changed position during the ITI as required. Success demonstrations introduced in Experiment 2 consisted of one actor manipulating a container for 5 s, opening it and emptying the contents into one hand. In experiment trials of Experiments 2–4, the actions of the two actors with their containers were similar in terms of tone and vigour. All sessions consisted of 12 experimental trials, across which A and B maintained their respective roles of attempter and helper or non-helper, according to the session condition. Type of session alternated (except in Experiment 4), with no more than one session per day, until a total of six sessions of each type were completed. In all experiments, the two actors played each role (A and B) in an equal number of sessions; in total three individuals served as actors. The frequency of selecting A versus B was compared using paired Student’s t -tests, and frequency of selecting each actor was compared against chance using one-sample t -tests; alpha was 0.05. Tests involving non-helper selections were two-tailed in Experiments 1 and 4, and one-tailed in Experiments 2 and 3 ( Table 1 ), as we predicted a bias against the non-helper following Experiment 1. Every trial was video recorded using a Sony HDD Handycam (Model No. DCR-SR220) mounted on a tripod and positioned between and slightly behind the two actors, providing an unobstructed view of the monkey in the test box. How to cite this article: Anderson, JR. et al . Third-party social evaluation of humans by monkeys. Nat. Commun. 4:1561 doi: 10.1038/ncomms2495 (2013).